Hybrid carbon nanotube yarn artificial muscle inspired by spider dragline silk Torsional artificial muscles generating fast, large-angle rotation have been recently demonstrated, which exploit the helical configuration of twist-spun carbon nanotube yarns. These wax-infiltrated, electrothermally powered artificial muscles are torsionally underdamped, thereby experiencing dynamic oscillations that complicate positional control. Here, using the strategy spiders deploy to eliminate uncontrolled spinning at the end of dragline silk, we have developed ultrafast hybrid carbon nanotube yarn muscles that generated a 9,800 r.p.m. rotation without noticeable oscillation. A high-loss viscoelastic material, comprising paraffin wax and polystyrene-poly(ethylene–butylene)-polystyrene copolymer, was used as yarn guest to give an overdamped dynamic response. Using more than 10-fold decrease in mechanical stabilization time, compared with previous nanotube yarn torsional muscles, dynamic mirror positioning that is both fast and accurate is demonstrated. Scalability to provide constant volumetric torsional work capacity is demonstrated over a 10-fold change in yarn cross-sectional area, which is important for upscaled applications. Artificial muscles are materials that generate a volume and/or shape change when stimulated [1] and have been variously configured to operate in a linear expansion/contraction mode; as bending cantilevers; and as torsionally rotating fibres or cylinders. Carbon nanotube (CNT) yarn operated as a rotating-type artificial muscle can generate over a thousand times larger rotation per muscle length [2] , [3] than previous torsional artificial muscles [4] , [5] , [6] . Torsional actuation and tensile contraction of a helically twisted CNT yarn are induced electrochemically [2] or by electrothermally, photothermally, thermally or chemically [3] caused volume changes of a guest that is confined within the yarn. Torsional actuation at an average 11,500 revolutions per minute results from Joule heating of a paraffin wax-filled, twist-spun CNT yarn [3] . Paraffin is a well-known thermal actuator material [7] , [8] , [9] in which the solid–liquid phase transition and thermal expansion provide ~30% volume expansion. When confined within the pore space between twist-spun CNT bundles, the wax volume increase drives a shortening and untwist of the host yarn that can be harnessed as tensile and torsional actuation, respectively. One way to physically understand the origin of torsional actuation (as well as tensile actuation) for the wax-containing CNT yarns is to note that twist-spun CNT yarns are most simply described as comprising a cascade of helical springs that are like ordinary metal springs, but made of CNTs. The helix bias angle ( α ) in the CNT yarns, which is the inclination angle between the CNTs and the helix axis, decreases with decreasing radial distance from the yarn centre. The approximate dependence of bias angle on yarn radius ( r ) is given by α =tan −1 (2 πrT ), where T is the inserted twist per yarn length. As shown in Fig. 1c , this helix angle for the outer yarn radius is small for the present yarns (compared with the bias angle of 54.73° that maximizes helix volume when the number of turns in the helix is kept constant [2] ). If the helical spring has a smaller bias angle than 54.73°, and the spring ends are tethered so that spring untwist cannot occur, then the spring contracts in length when spring volume increases [2] . Hence, when the guest in the thermally powered muscle expands due to heating, the yarn’s bias angle increases to thereby produce contraction in yarn length, by an amount that is affected by whether or not torsional actuation is allowed. 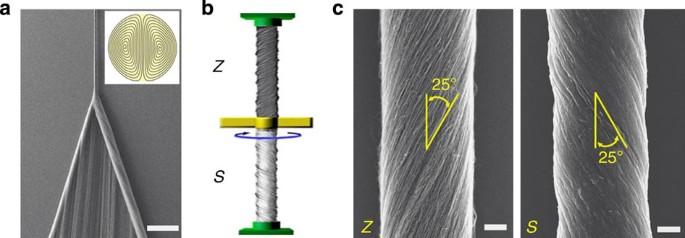Figure 1: Fabrication and configuration of hybrid yarn for torsional actuation. (a) SEM image of dual Archimedean-type twist insertion during spinning from a CNT forest. The inset illustrates a dual Archimedean scroll. Scale bar, 500 μm. (b) Schematic illustration of muscle configurations and yarn structures for torsional actuation. The paddle is located in the middle of a two-end-tethered, half-infiltrated, heterochiral yarn. The arrow indicates the observed direction of paddle rotation during reversal of thermal actuation for aSyarn filled with the poly(ethylene–butylene)-polystyrene (SEBS) mixture with paraffin wax. The green supports at yarn ends are tethers that prohibit end rotation. (c) SEM images of unfilled CNT yarn (Zchirality) and wax-SEBS-infiltrated CNT yarn (Schirality). The average diameter ofSandZyarn is ~20 μm. The average bias angle is~25°. Scale bars, 5 μm. Figure 1: Fabrication and configuration of hybrid yarn for torsional actuation. ( a ) SEM image of dual Archimedean-type twist insertion during spinning from a CNT forest. The inset illustrates a dual Archimedean scroll. Scale bar, 500 μm. ( b ) Schematic illustration of muscle configurations and yarn structures for torsional actuation. The paddle is located in the middle of a two-end-tethered, half-infiltrated, heterochiral yarn. The arrow indicates the observed direction of paddle rotation during reversal of thermal actuation for a S yarn filled with the poly(ethylene–butylene)-polystyrene (SEBS) mixture with paraffin wax. The green supports at yarn ends are tethers that prohibit end rotation. ( c ) SEM images of unfilled CNT yarn ( Z chirality) and wax-SEBS-infiltrated CNT yarn ( S chirality). The average diameter of S and Z yarn is ~20 μm. The average bias angle is~25°. Scale bars, 5 μm. Full size image If an ordinary metal spring having a bias angle far below 54.73° is stretched, the volume of the spring decreases and rotation generally occurs between spring ends, unless the spring is tethered to prevent such rotation. The wax-containing twist-spun yarns operate analogously, but in the inverse direction during thermal actuation. Thermal expansion of the wax or wax/polymer composite within the yarn causes the yarn volume to increase, the yarn length to contract and the yarn to untwist to provide torsional actuation. This description assumes that the string length (that is, the wire length or the nanotube length) within the helical spring is invariant, which is a good approximation. If a helical spring with constant string length is forced to increase volume without length change, the simple geometry of a helix indicates that the spring must untwist, which is what we observe for thermal expansion of the wax-containing CNT yarns, independent of whether tensile actuation is allowed. More detailed analysis of the relationship between CNT yarn volume change and torsional and tensile actuation has been previously provided [2] , [3] . Fast heating of wax-filled CNT yarns using square-wave electrical pulses produces impressive contraction rates and torsional rotation speeds. However, mechanical oscillation complicates control of the torsional and tensile actuation stroke when fast actuator response is required. Spider dragline silk, which is used as a lifeline and for the web’s outer rim and spokes, has exceptional strength and toughness [10] . Especially interesting for the present work, this dragline silk dampens torsional rotations, thereby preventing the spider from rotating uncontrollably. This silk comprises a block copolymer in which alanine blocks form crystalline domains that are connected by amorphous glycine blocks [11] . The alanine blocks provide stiffness, so that return to the starting orientation occurs, and the amorphous blocks provide mechanical energy loss, so that oscillations about the starting torsional orientation are quickly damped. Spider-silk-like damped dynamic behaviour in torsional actuators would help minimize unwanted dynamic oscillations [12] , thereby improving positional control and decreasing the response time needed to achieve final torsional position. The present research aim is to realize biomimetic torsional artificial muscles by optimal design of the guest material in twist-spun CNT yarns. We synergistically combine the large thermally induced volume changes provided by paraffin wax with mechanical dampening that arises from the mixtures of this wax with a triblock copolymer. We build upon previous work that showed large peaks in mechanical dampening occur near the wax melting temperature for specific CNT-free mixtures of paraffin wax with polystyrene-poly(ethylene–butylene)-polystyrene (SEBS) triblock copolymer that have been used as shape memory elastomers [13] . SEBS is a classical phase-separating block copolymer, with a polystyrene (PS)-rich phase dispersed within the elastomeric ethylene–butylene (EB) continuous phase. Paraffin wax that is added to the SEBS forms crystalline domains. For low paraffin wax content, small crystal-size paraffin is confined to the EB regions [13] . For paraffin levels above 50 wt%, the excess wax is no longer completely confined within the EB regions. This dependence of guest morphology on wt% paraffin wax affects mechanical dampening and provides a maximum in dampening coefficient at a 8:2 weight ratio of wax:SEBS. Herein, we combine mixtures of wax and SEBS as guest materials within CNT yarns and investigate their dynamic torsional actuation. The peak rotation speed realized without noticeable oscillation was ~9,800 r.p.m. for a hybrid yarn containing 8:2 wax-SEBS yarn guest when excited by a 0.5 Hz square-wave voltage. Hybrid yarn muscle fabrication The presently used configuration for torsional actuation has the CNT yarn under tensile load, tethered at both ends, and one-half-infiltrated with the wax-SEBS guest [3] . One-half of the yarn length had left-hand inserted twist ( Z -type) and the opposite half had right-hand inserted twist ( S -type). This heterochiral configuration provides highly reversible torsional actuation only because the structural rigidity of the SEBS polymer prevents cancelation of S and Z twist. The rotor was attached at yarn midpoint, between the S and Z yarn segments. Twist-spun, dual Archimedean scroll yarns were used to prepare the torsional muscles. A single sheet of carbon multiwalled nanotubes (MWNTs) was drawn from a MWNT forest and twist spun using ~228 turns per cm of inserted twist to form an ~20 μm diameter yarn ( Fig. 1a ). A blend of SEBS elastomer and a paraffin wax (melting at ~53 to 57°) was infiltrated into the yarn by dipping one-half of a MWNT yarn in a toluene solution of SEBS and paraffin. Following removal of the yarn from the infiltration bath and solvent evaporation, the unfilled portion of the yarn was completely untwisted by attaching one end to an electric motor and then re-twisted to the opposite chirality and the same inserted twist by reversing the motor direction. The final CNT composite yarn with the infiltrated segment of S chirality joined to the unfilled segment of Z chirality is shown in Fig. 1b . The overall scheme used for fabrication of the hybrid yarn is described in Supplementary Fig. 1 . Scanning electron microscopy images show a wax-SEBS-infiltrated S segment and non-infiltrated Z segment having the same bias angle of 25° ( Fig. 1c ). Unless otherwise indicated (such as for the experiments pertaining to muscle scalability), the reported experiments utilize the yarns and muscle configuration described in this paragraph. To evaluate torsional actuation, the hybrid yarn was tethered at both yarn ends under fixed tensile load (~0.35 MPa) and a Mylar paddle was attached at yarn midpoint. The sample was heated electrothermally by applying a square-wave voltage. The experimental method used to characterize torsional actuation is more completely described in Supplementary Fig. 2 . Electrothermally powered reversible and tunable torsional actuation As for our previous torsional wax-filled CNT muscles [3] , electrothermally driven expansion of the wax-SEBS in the guest-containing yarn segment caused untwist of this segment. The hydraulic pressure generated by the expanding guest acts against the CNT bundles and their high stiffness and helical orientation favours anisotropic yarn volume expansion by radial expansion, axial contraction and partial CNT untwist. Guest material, even in the molten state, does not tend to exude from the yarn interior due to the unfavourable surface energy thermodynamics. During thermally produced expansion of the guest-filled yarn segment, this segment untwists, which causes untwist of the guest-free yarn segment having opposite chirality. Since the guest in the guest-filled yarn segment does not completely melt during thermal actuation, the unmelted guest acts as an internal return spring that allows the paddle to return to the starting rotation angle when torsional actuation is reversed by guest cooling and subsequent contraction. In this study, the dependence of guest morphology on wt% paraffin wax affects mechanical dampening both for previously studied CNT-free shape memory rubber and for the presently investigated composite of wax-SEBS in a CNT host. We surprisingly find ( Fig. 2a ) that the maximum in loss tangent (tan δ occurs for the CNT composite at the same 8:2 weight ratio of wax:SEBS as previously found for CNT-free wax-SEBS composite. 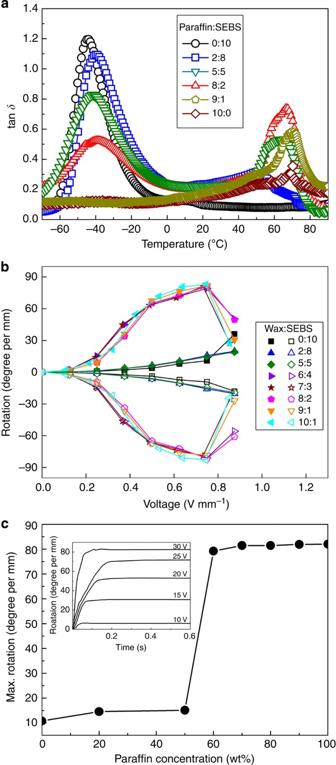Figure 2: Reversible and tunable torsional actuation. (a) Measured loss tangent (tanδ) as a function of temperature for CNT yarns containing various wt% ratios of paraffin to poly(ethylene–butylene)-polystyrene (SEBS). The tanδpeak around −40 °C corresponds to the phase transition temperature of soft ethylene–butylene segments in SEBS, and the tanδpeak around 60 °C corresponds to the phase transition temperature of the paraffin wax. (b) Thermal torsional actuation for various wax-SEBS-infiltrated yarn versus applied voltage for a 0.5 Hz square-wave voltage using 50% duty cycle. Voltage pulse measurements of maximum torsional angle of untwist on increasing voltage pulse from previous measurements (filled symbols) and on decreasing pulse voltage from previous measurements (open symbols) are designated using different arbitrarily chosen signs for the twist angle in order to avoid overlap of data. (c) The equilibrium maximum torsional rotation angle as a function of the wt% of paraffin wax in the yarn guest, when powered using 30 V (0.75 V mm−1). Inset: torsional rotation angle as a function of time for various voltage inputs for 8:2 wax-SEBS yarn guest. Figure 2: Reversible and tunable torsional actuation. ( a ) Measured loss tangent (tan δ ) as a function of temperature for CNT yarns containing various wt% ratios of paraffin to poly(ethylene–butylene)-polystyrene (SEBS). The tan δ peak around −40 °C corresponds to the phase transition temperature of soft ethylene–butylene segments in SEBS, and the tan δ peak around 60 °C corresponds to the phase transition temperature of the paraffin wax. ( b ) Thermal torsional actuation for various wax-SEBS-infiltrated yarn versus applied voltage for a 0.5 Hz square-wave voltage using 50% duty cycle. Voltage pulse measurements of maximum torsional angle of untwist on increasing voltage pulse from previous measurements (filled symbols) and on decreasing pulse voltage from previous measurements (open symbols) are designated using different arbitrarily chosen signs for the twist angle in order to avoid overlap of data. ( c ) The equilibrium maximum torsional rotation angle as a function of the wt% of paraffin wax in the yarn guest, when powered using 30 V (0.75 V mm −1 ). Inset: torsional rotation angle as a function of time for various voltage inputs for 8:2 wax-SEBS yarn guest. Full size image Figure 2b shows the dependence of rotation angle on applied voltage for identically prepared CNT yarns containing yarn guest having different relative concentrations of wax and SEBS copolymer. The maximum rotation angle ( Fig. 2c ) dramatically increases from ~15 to ~80° mm −1 in the concentration range between 50 and 60 wt% of paraffin wax in the wax-SEBS guest. This maximum rotation, corresponding to untwist of the actuating yarn segment, was ~0.97% of the inserted twist. The data show little dependence on paraffin wt% at both lower and higher paraffin concentrations. Interestingly, this transition in maximum torsional rotation occurs for paraffin levels (above 50 wt%) where transmission electron microscopy indicates a transition from wax completely confined within rubbery EB regions of the copolymer to a structure in which excess wax is no longer localized within this polymer block [13] . Based on this relationship between transition in maximum torsional actuation and structure change, it appears that nanocrystalline wax within the EB regions contributes little to the changes in guest volume that drives torsional actuation. The dependence of rotation angle on applied voltage ( Fig. 2b ) is complex and dependent on guest composition. In all cases, however, rotation angle was substantially identical for measurements taken on increasing and decreasing voltage pulse amplitude. This lack of dependence on prior history will be useful for practical applications of the yarn torsional muscles. Since yarn electrical resistance is largely temperature independent ( Supplementary Fig. 3 ) for the range of investigated applied voltages ( V ), Joule heating should be proportional to V 2 . Hence, the dependence of rotation angle on applied voltage would be approximately quadratic if yarn volume increased linearly with temperature ( Fig. 2b ). In fact, the effective average thermal expansion coefficient for paraffin waxes above room temperature in the solid state (including volume changes due to phase transitions) is much larger than in the liquid state [3] . Consequently, yarns containing high relative wax concentrations (wax:SEBS ratios ≥6:4) show a smaller increase of rotation angle with voltage change in the liquid state, where V is high, than in the solid state, where voltage is low. Moreover, for these yarns containing high wax concentrations, the rotation angle actually decreases with increasing voltage per actuator length for applied voltages above 0.75 V mm −1 ( Fig. 2b ). This decrease is not due to permanent evaporative loss of wax from the actuating yarn segment, since decreasing actuation pulse voltage results in the same dependence of rotation angle on pulse voltage as for increasing pulse voltage. The origin of this decrease in rotation angle at high temperatures appears to be reversible extrusion of the paraffin wax from the interior of the actuating yarn when the hydraulic energy associated with guest expansion exceeds the surface tension-related confinement energy. These mechanisms are also supported by observed smaller rotation and monotonically increasing rotation with increasing temperature in yarns containing low wax concentrations (wax:SEBS ratios of ≤5:5). This latter result is reasonable because of the lower thermal expansion coefficient for the SEBS compared with paraffin wax and the lack of fluidity for SEBS at all relevant temperatures. These factors combine to prohibit guest extrusion from the yarn and limit volume expansion, thereby giving small, monotonically increasing rotation with increasing voltage. 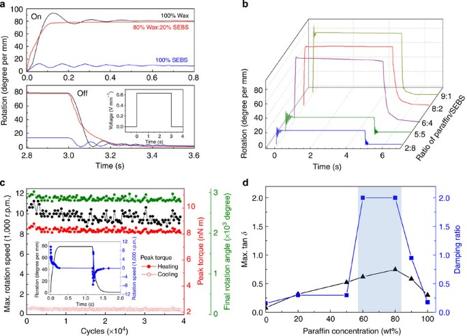Figure 3: Damped torsional actuation: (a) Torsional rotation versus time for hybrid yarn artificial muscles that are powered using the square-wave voltage input that is shown in the inset. The plots are for when the drive voltage is turned on (top) and turned off (bottom). The wt% ratios of wax to poly(ethylene–butylene)-polystyrene (SEBS) in the yarn guest for the different investigated muscles are as follows: 100% wax (black line), 80% wax (red line), and 0% wax (blue line). (b) Torsional rotation versus time forS-Zyarns (containing paddle at yarn center) that are one-half-infiltrated with various weight ratios of paraffin to SEBS. (c) Maximum rotation speed (black solid circles), final rotation angle (green solid circles), and the magnitude of peak torque (red solid circles) versus cycle number for a hybrid yarn containing 8:2 wax-SEBS yarn guest, when excited by a 0.5 Hz square-wave voltage to 0.63 V mm−1using 50% duty cycle. The red open circles provide the magnitude of peak torque during the cooling part of the torsional actuation cycle. Inset: rotation angle (black solid line) and rotation speed (blue solid circle) versus time for one complete cycle. The peak rotation speed was ~9,800 revolutions per minute. (d) The maximum high temperature damping loss coefficient tanδand the damping ratio for torsional relaxation on torsional oscillations as a function of wt% paraffin wax in the wax-SEB mixture within the hybrid yarn muscle. The blue area indicates the wt% of wax where over-dampened torsional response is obtained. Figure 3a shows the dependence of torsional rotation on time during forward and reverse actuation driven by a 0.167 Hz square-wave voltage (between 0 and 0.63 V mm −1 , with 50% duty cycle). These data indicate that an 8:2 wax-SEBS weight ratio results in actuation that is substantially free of oscillation for both the forward and reverse actuation processes. In general the rates of forward actuation by joule heating and reverse actuation by environmental cooling will differ, and depend upon volumetric power input to the yarn for forward actuation and yarn diameter for reverse actuation. As shown in Fig. 3b , for additional guest compositions and different square-wave drive voltage, support this conclusion. The torsional rotation was produced by a 0.75 V mm −1 voltage pulse that was 5-s long. These results show that torsional overdamping occurs to largely eliminate torsional oscillations for wax-SEBS ratios of 6:4 and 8:2. Spider dragline silk-like dampening results in the range between these weight fractions. For lower (5:5 and 2:8) or higher (9:1) weight fraction of paraffin wax, torsional oscillations occur (due to underdampening), which are particularly pronounced during the heating step. Figure 3: Damped torsional actuation: ( a ) Torsional rotation versus time for hybrid yarn artificial muscles that are powered using the square-wave voltage input that is shown in the inset. The plots are for when the drive voltage is turned on (top) and turned off (bottom). The wt% ratios of wax to poly(ethylene–butylene)-polystyrene (SEBS) in the yarn guest for the different investigated muscles are as follows: 100% wax (black line), 80% wax (red line), and 0% wax (blue line). ( b ) Torsional rotation versus time for S-Z yarns (containing paddle at yarn center) that are one-half-infiltrated with various weight ratios of paraffin to SEBS. ( c ) Maximum rotation speed (black solid circles), final rotation angle (green solid circles), and the magnitude of peak torque (red solid circles) versus cycle number for a hybrid yarn containing 8:2 wax-SEBS yarn guest, when excited by a 0.5 Hz square-wave voltage to 0.63 V mm −1 using 50% duty cycle. The red open circles provide the magnitude of peak torque during the cooling part of the torsional actuation cycle. Inset: rotation angle (black solid line) and rotation speed (blue solid circle) versus time for one complete cycle. The peak rotation speed was ~9,800 revolutions per minute. ( d ) The maximum high temperature damping loss coefficient tan δ and the damping ratio for torsional relaxation on torsional oscillations as a function of wt% paraffin wax in the wax-SEB mixture within the hybrid yarn muscle. The blue area indicates the wt% of wax where over-dampened torsional response is obtained. Full size image The time required for achieving equilibrium rotation will depend upon whether the yarn is underdamped, critically damped, or overdamped. Critically damped systems quickly reach the equilibrium position without overshoot and oscillation when a step change in stimulus occurs. Overdamping shows a slower response than that of critical damping and also without oscillation. Underdamped systems will overshoot the equilibrium position and gradually oscillate with decreasing amplitude to reach a stable equilibrium. For fast positioning and oscillation-free torsional actuation, strong damping, preferably critical damping, is required. Comparison of the torsional rotation in wax-only and SEBS-only filled yarns for the same square-wave drive voltage and the same configuration of the torsional muscle show both to be underdamped, but with a shorter time to the first oscillation peak with SEBS as guest. Under identical test conditions, the rate of torsional actuation will be dependent upon the average heat capacity of the guest. Since the electrical input power is constant and it takes more energy to heat the paraffin wax (which is used to store thermal energy) than is needed to heat SEBS to the same temperature ( Fig. 3a ), the longer response time for the 100% wax yarn is understandable. The time response for the optimal 8:2 wax-SEBS ratio yarn in Fig. 3a suggests that this yarn is not severely overdamped. At the time (0.13 s) where the 100% wax yarn has reached its first oscillatory maximum (at a 15° mm −1 higher rotation angle than for static equilibrium), the 8:2 wax-SEBS ratio yarn is already within 1° mm −1 of the rotation angle for static equilibrium. A severely overdamped yarn would be significantly retarded in the initial rotation rate in comparison to the underdamped yarn. Figure 3b results (using a higher input power) indicates that about the same time (0.4 s) is needed to realize near-equilibrium rotation for the 6:4 and 8:2 wax-SEBS ratio yarns, thereby providing further evidence that the 8:2 wax-SEBS yarn is not severely overdamped. The overdamped behaviour for the SEBS-paraffin filled yarn permits the rapid stabilization of the torsional rotation after the voltage is applied. In contrast, the continued paddle oscillation with slow decay in the paraffin-only filled yarn requires an order of magnitude longer time for a stable rotation to occur. The high damping efficiency of the SEBS-paraffin guest is related to mixed phase state of the heated guest consisting of molten paraffin and the rubbery EB phase with hard segment (PS) of SEBS each playing a role in mechanical energy absorption to inhibit oscillation and quickly reach a stable state. The remarkable difference in the damping of torsional actuation in hybrid yarns having different wax-SEBS ratios (8:2 and 2:8) are shown in Supplementary Movie 1 . Fast, reversible torsional actuation was demonstrated for the 20-μm-diameter yarn filled with an 8:2 weight ratio of wax-to-SEBS, which rotated a 25 times heavier paddle at yarn midpoint ( Fig. 3c ). To determine the long-term stability and reversibility of torsional actuation, we conducted 40,000 continuous actuation cycles for this yarn muscle and analysed torsional actuation in terms of maximum rotation speed, peak torque and final rotation angle for every 400th cycle to provide the result for Fig. 3c , which are discussed in the following paragraphs. These results were obtained for 4-cm-long actuating yarn weighing ~3.2 μg, which was electrothermally powered by a 0.5 Hz, 0.63 V mm −1 , square-wave voltage using 50% duty cycle. The torsional rotation angle on heating was stable at ~2,850 degrees, or ~71° mm −1 relative to total yarn length (the inset of Fig. 3c ), and is fully reversed on cooling and similar in magnitude to the 64° mm −1 rotation reported previously for paraffin/MWNT yarns [3] . The peak rotation speed was ~9,800 r.p.m., compared with a maximum average rotation speed of 11,500 r.p.m. for a paraffin/MWNT yarn. The gravimetric torque generated by rapidly heating the above yarn by using square-wave electrical pulses was comparable with those of large electric motors. The peak torque ( τ p = αI ) shown in Fig. 3c was estimated from the observed initial paddle acceleration ( α ) and paddle moment of inertia ( I = ml 2 /12=1.6 × 10 −13 kg m −2 , where l is one-half the paddle length and m is the paddle mass). The peak torque during heating was much higher than on cooling. Little variation in these torques were observed over the investigated ~40,000 cycles ( Fig. 3c ). Similarly, the average torque applied by the yarn during the heating cycle could be determined from the final paddle rotation and heating period as 8.29 nN m. The average gravimetric torque is 2.21 N m kg −1 for the actuating yarn mass of 3.2 μg. A strong correlation exists between the magnitude of the paraffin-melting induced tan δ peak and the damping response during torsional actuation of wax-SEBS filled MWNT yarns ( Fig. 3d ). The blue area of Fig. 3d indicates stable torsional behaviour, with overdamping providing an ~2 damping ratio (as obtained from the ratio of successive rotation angle peak heights shown in the Supplementary Fig. 4 and Supplementary Note 1 ). Scalability of muscle diameter to provide greatly increased muscle torque, without sacrificing specific work capacity, is important for extending the range of application possibilities for these CNT hybrid torsional muscles. We demonstrate this scalability by characterizing torsional actuation for muscles that are structurally analogous (since they have the same bias angle and the same yarn guest), but have very different diameters (67, 140 and 220 μm). Yarns containing S and Z segments of equal length were obtained by inserting twist into the midpoint of a forest-drawn sheet stack, where the yarn diameter was determined by the number of sheets in the sheet stack. After inserting twist until a bias angle ~27° was obtained for each muscle segment, both segments were infiltrated with 8:2 wax:SEBS yarn guest. A paddle attached at yarn midpoint, which was used to enable the initial twist insertion, was deployed for torque measurement. Torque was then directly obtained as a function of static applied electrical power by measuring the force that this paddle applied to a microbalance when the torsional muscle was actuated ( Fig. 4a ). 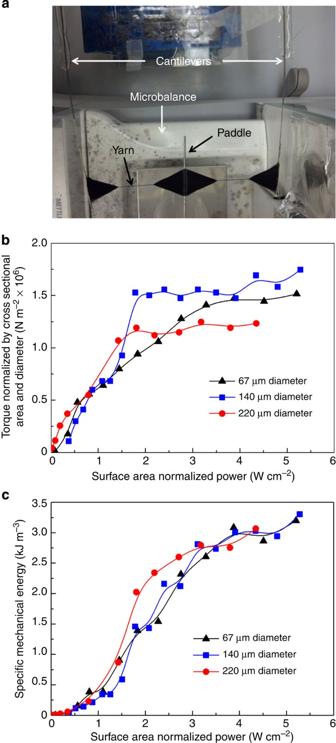Figure 4: Measurement apparatus and results for the scalability of torsional actuation. (a) Photograph of measurement configuration for torque measurements using a microbalance. (b) Static torque versus surface-area-normalized applied electrical power for 67, 140 and 220 μm diameter, fully infiltrated, heterochiral yarns, all with bias angles of ~27°. (c) Torsional work density for these yarn muscles versus applied electrical power normalized to muscle surface area, calculated as one-fourth the product of the measured static torque and the measured rotation angle for zero external torque. This method of calculating volumetric energy density approximates the maximum possible energy density obtainable for a muscle where torque linearly depends on rotation angle. Figure 4: Measurement apparatus and results for the scalability of torsional actuation. ( a ) Photograph of measurement configuration for torque measurements using a microbalance. ( b ) Static torque versus surface-area-normalized applied electrical power for 67, 140 and 220 μm diameter, fully infiltrated, heterochiral yarns, all with bias angles of ~27°. ( c ) Torsional work density for these yarn muscles versus applied electrical power normalized to muscle surface area, calculated as one-fourth the product of the measured static torque and the measured rotation angle for zero external torque. This method of calculating volumetric energy density approximates the maximum possible energy density obtainable for a muscle where torque linearly depends on rotation angle. Full size image The torque, normalized to the yarn’s cross-sectional area and diameter D ( Fig. 4b ), is plotted as a function of applied voltage/yarn surface area, which should correlate with yarn temperature for these different diameters torsional muscles. These results provide evidence that yarn torque is proportional to D 3 . The relatively minor differences between results for different diameter yarns can be a result of slight variation in the amount of wax:SEBS infiltrated, minor differences in the yarn bias angle, and subtle difference in yarn structure caused by the need to fabricate increasing diameter yarns from increasing number of stacked sheets. Most important, by also measuring the torsional stroke and multiplying it by the torque, the mechanical output energy of the yarn is shown to almost perfectly scale with yarn volume ( Fig. 4c ), despite yarn cross-sectional area and yarn torque spanning ranges of over an order of magnitude and a factor of 35, respectively. Physical insight into this scalability results from the following considerations ( Supplementary Note 2 ). Use of the same bias angle for all yarns implies structural similarity. From the above described equation that α =tan −1 ( πDT ), obtaining the same bias ( α ) for all yarns required twist insertion per yarn length ( T ) that inversely depends on the yarn diameter ( D ). The above obtained structural similarity implies similar torsional stroke in turns per meter, when normalized to the inverse of fibre diameter. Furthermore, increasing the diameter of a yarn increases the cross-sectional area by a factor of diameter squared, while simultaneously increasing the lever arm by a factor of diameter, to yield a torque proportional to D 3 . The product of this torque and torsional stroke determines the mechanical output energy which, as expected for a perfectly scalable actuator, increases with yarn volume (diameter squared times length). Electrothermally actuated torsional mirror array Hybrid torsional muscles were applied to actuate a mirror array. As shown in Fig. 5a , torsional muscle yarn was suspended between two connection posts and a 3 mm × 3 mm square mirror attached at yarn midpoint. Voltage applied to the two posts electrothermally actuated and rotated the yarn and attached mirror. The angle of mirror rotation was controllable ( Fig. 5b ) and fast 90° switching between horizontal and vertical mirror angles was demonstrated using 0.34 V mm −1 at 0.5 Hz ( Supplementary Movie 2 ). The fast rotation and overdamped response gave non-oscillatory rotation within 0.13 s allowing refresh rates of 0.5 Hz ( Fig. 5c ). In the demonstrated example, each mirror acts as a single pixel in a simple binary image display with mirror pixels determined by ‘on’ and ‘off’ rotation angle as shown by the photographs in Fig. 5b . 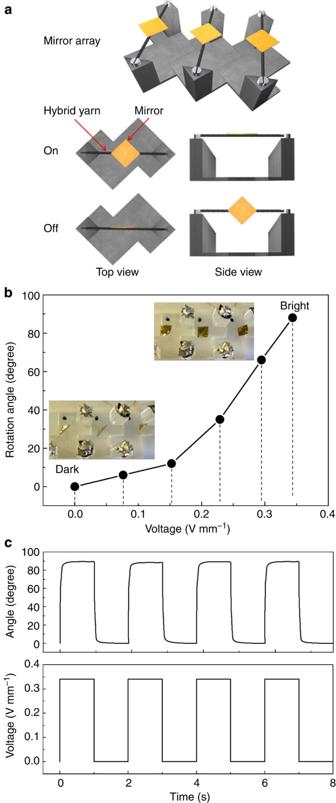Figure 5: Electrothermally actuated torsional mirror array. (a) Schematic illustration of the demonstrated use of torsional yarn muscle to precisely rotate mirrors without producing significant torsional oscillations. The torsional yarn muscle was suspended between two posts and a 3 mm × 3 mm square mirror was attached at yarn midpoint. Voltage applied to the two posts electrothermally actuated the yarn to produce torsional rotation of the attached mirror. Three actuating mirrors were assembled and simultaneously switched from mirror tilt at 90° inclination with respect to the horizontal direction (voltage off) to 0° inclination (voltage on). (b) Mirror rotation angle versus applied voltage is shown. ‘Dark’ image corresponding to mirrors in the voltage off state, and ‘bright’ image corresponding to mirrors in the voltage on state (although the surface reflectivity of the substrate and inadequate mirror reflectivity interferes with the visual appearance). (c) The time dependence of torsional rotation of the mirror (top) is compared with the time dependence of the applied voltage (bottom). The applied square-wave voltage was 0.34 V mm−1at 0.5 Hz. Figure 5: Electrothermally actuated torsional mirror array. ( a ) Schematic illustration of the demonstrated use of torsional yarn muscle to precisely rotate mirrors without producing significant torsional oscillations. The torsional yarn muscle was suspended between two posts and a 3 mm × 3 mm square mirror was attached at yarn midpoint. Voltage applied to the two posts electrothermally actuated the yarn to produce torsional rotation of the attached mirror. Three actuating mirrors were assembled and simultaneously switched from mirror tilt at 90° inclination with respect to the horizontal direction (voltage off) to 0° inclination (voltage on). ( b ) Mirror rotation angle versus applied voltage is shown. ‘Dark’ image corresponding to mirrors in the voltage off state, and ‘bright’ image corresponding to mirrors in the voltage on state (although the surface reflectivity of the substrate and inadequate mirror reflectivity interferes with the visual appearance). ( c ) The time dependence of torsional rotation of the mirror (top) is compared with the time dependence of the applied voltage (bottom). The applied square-wave voltage was 0.34 V mm −1 at 0.5 Hz. Full size image The system can be readily scaled to multimirror arrays for a simple, low cost binary display for signage. Electrothermal yarn torsional actuation can also achieve a controlled mirror rotation to realize simple and accurate laser positioners. The mechanisms of mechanical energy dissipation in the hybrid yarns have been investigated using dynamic mechanical analysis. The tan δ so obtained is the ratio of loss modulus to storage modulus and provides a measure of energy dissipated to energy stored during dynamic deformation [14] . As shown in the Fig. 2a , tan δ is strongly temperature dependent and one tan δ peak is seen in the 100% SEBS yarn between −70 °C and 90 °C, whereas all hybrid yarns show two distinct tan δ peaks. All measurements were conducted with 1 Hz frequency. Low temperature peaks around −40 °C correspond to the relaxation of EB segments. The higher peak at ~60 °C is attributed to the solid–liquid phase transition of paraffin [13] , since our paraffin melts at 53~57 °C. As we previously mentioned, the maximum in tan δ at the 8:2 weight ratio of wax:SEBS confirms the dominance of the wax-SEBS guest in determining the viscoelastic properties of the hybrid yarn. It is likely that the molten paraffin provides the fluid-like viscous response at and above its melting temperature. The elasticity of the guest material is provided by the SEBS component. Enhanced damping occurs when both viscous and elastic mechanical elements are active. With insufficient paraffin, the guest acts as a low-loss elastomer. With high levels of paraffin, there is insufficient SEBS to retard the elastic response and again, the energy dissipation is reduced. As a consequence, high damping in hybrid yarn torsional muscles occurs with guest materials having the optimal blend of paraffin and SEBS elastomer ( Fig. 3a ). Using the viscoelastic blend of paraffin wax and SEBS copolymer, it is possible to operate highly reversible torsional actuation with overdamping and rapid positioning. With the optimal ratio of paraffin wax and SEBS, we can obtain large and fast rotations, high reversibility and high stability (overdamped) torsional artificial muscles driven by the melting and volume expansion of paraffin incorporated with SEBS. We can control the torsional damping during torsional actuation near the melting transition of paraffin by confinement of paraffin in EB segments of SEBS. Such hybrid yarn artificial muscles have the advantage of precise and rapid positioning, which is essential for some applications, such as the demonstrated micromirror arrays. The present demonstration of muscle scalability, especially when combined with actuator positional control using spider-inspired torsional dampening, dramatically expands the range of applications possibilities for twist-spun CNT torsional muscles. This scalability means, for example, that large mirrors, shutters and pixels for displays can be rotated for optical applications. Like for all thermal or electrical artificial muscles, upscaling artificial muscle diameters decrease muscle response rate. Torsional pumps based on the described torsional muscles could be upscaled in power densities by using the cooling capacity of the pumped liquid to accelerate the cooling needed to reverse actuation. On the other hand, the scalability of torsional actuation may be especially important for application where neither slow response rate nor mechanical oscillations are problems, like when low ambient temperature changes or photothermally produced temperature changes drive torsional actuation for control purposes or for harvesting low-grade thermal energy. However, at least in the near term, relatively small diameter torsional muscles are most likely to be deployed, such as for controlling valves in microfluidic chips, controlling fuel delivery for engines of diverse sizes (using fluidic amplifiers and fluidic logic circuits), and enabling torsional rotation for minimally invasive surgery, where fast response without torsional oscillations are desirable. For such applications, the hereby provided ability to precisely control torsional actuation by using the spider-inspired approach is especially noteworthy, other torsional artificial muscles in the literature provide at least a thousand times lower torsional rotation per muscle length and are hysteretic, which means that positional control is challenging. Ordinary electric motors cannot be downsized without dramatic decrease in power-to-weight capabilities [15] , which is not the case for our torsional motors. Moreover, the presently demonstrated ability to dampen undesired end of stroke oscillations directly enables such dampening of tensile oscillations, since tensile and torsional oscillations are coupled. Materials SEBS copolymer with styrene/ethylene–butylene ratio of 29:71 and commercial paraffin wax with melting point of 53~57 °C were obtained from Sigma-Aldrich (#200557 and #327204, respectively). Paraffin waxes are crystalline in the solid state with a thermal expansion coefficient of a few hundred parts per million per degree centigrade and exhibit a volume expansion of 10–20% when melted [16] . CNT yarn fabrication and structure The first procedure in making a hybrid yarn artificial muscle is to twist-spin a yarn from nanotubes drawn from a CNT forest [17] , [18] . Briefly, multiwalled CNT (MWNT) forests that are drawable to produce sheets were grown by the catalytic reaction of acetylene (C 2 H 2 ) over an iron catalyst at 700 °C in an Ar/H 2 atmosphere. The growth substrate was a silicon wafer coated with a 1–3-nm thick iron catalyst layer by e-beam evaporation. This substrate was placed into a 3-inch diameter quartz tube furnace that had been heated to 700 °C in a mixture of 750 s.c.c.m. Ar and 100 s.c.c.m. H 2 . After a 5-min residence time at oven temperature, MWNT forests were grown in 2 to 5 min after introduction of 50 s.c.c.m. of C 2 H 2 to this gas mixture. The utilized MWNT forests are ~400 μm length having an outer diameter ( d ) of ~12 nm and ~9 walls. Symmetric twist insertion during sheet draw from a forest and for a pre-drawn nanotube sheet suspended between rigid supports provides dual Archimedean structure [17] . Approximately ~228 turns per cm were necessary to collapse a 11-cm-long sheet into a 7-cm-long yarn having dual Archimedean scroll structure. The yarn diameter was controlled to ~20 μm by fixing the drawn forest width at ~1 cm. Multiple sheets were stacked before twist insertion in order to obtain the larger diameter yarns used for the demonstration of scalability in torsional muscle performance. Fabrication of hybrid yarn artificial muscle A commercially purchased paraffin wax and SEBS elastomeric copolymer were dissolved in toluene at various ratios. Paraffin wax-SEBS half-infiltrated yarn muscles were typically fabricated using simple infiltration method, where a two-end-tethered twist-spun yarn was half immersed in the wax-SEBS solution for 24 h at 60 °C. The yarn was removed from the composite solution and the solvent was completely evaporated at room temperature. Then, the unfilled S- type yarn was untwisted and re-twisted to Z -type by a motor attached at one end. In this way, the heterochiral (with equal length segments having opposite chirality) half-infiltrated yarn was obtained. The linear combination of actuating yarn segments having opposite chirality (designated Z and S yarn), with paddle placed at their interconnection, is predicted to maximize initial rotation of the paddle [2] . The chirality and morphology of nanotube yarn muscles were investigated by field emission scanning electron microscopy (Hitachi, S4800). Electrically powered actuation measured by thermomechanical analysis To investigate the torsional actuation, a 4-cm-long, half-infiltrated, and heterochiral dual Archimedean yarn was tethered at both ends in a thermal mechanical analyser (TMA) (TMA, SEIKO TMA/SS7100) as shown in Supplementary Fig. 2 . Each clamped yarn end was connected to a platinum wire using silver paste and then contacted to the voltage SourceMeter (Keithley 2635) after complete drying of the silver paste. To operate the hybrid yarn actuator, a constant tensile stress of 0.35 MPa was applied by the TMA and the sample excited by a 0.5 Hz square-wave voltage using 50% duty cycle. The tensile actuation was monitored using TMA. The rotation angle (degree per mm) of the plastic paddle attached at yarn midpoint was precisely observed and analysed by a high-speed imaging camera with high resolution (2,000 frame/s, Phantom Miro eX2). Damping loss factor by using dynamic mechanical analysis A Perkin Elmer instrument was used for obtaining loss tangent (tan δ =E′′/E′) from storage modulus (E′) and loss modulus (E′′). The yarn tested by dynamic mechanical analysis (DMA) was 5 mm in length. The yarn samples were cooled to –70 °C and measured during heating from –70~90 °C with 5 °C min −1 rate. An oscillation of 1 Hz was applied continuously. The hybrid yarn was mounted vertically in the DMA and operated in the environment of dry nitrogen purged at 50 ml min −1 . Mirror device fabrication Torsional muscle yarn was suspended between two connection posts and a 3 mm × 3 mm square mirror attached at yarn midpoint. Voltage applied to the two posts electrothermally actuated and rotated the yarn and attached mirror. The binary image of the assembled mirror pixels was determined by the ‘on’ and ‘off’ voltage states. The rotation of mirrors was conducted by a square-wave voltage of 0.34 V mm −1 . The mirrors were rotated in one of the two states (that is, 0 degree for voltage off and 90 degree for voltage on). How to cite this article : Chun, K.-Y. et al. Hybrid carbon nanotube yarn artificial muscle inspired by spider dragline silk. Nat. Commun. 5:3322 doi: 10.1038/ncomms4322 (2014).